Oxidation-assisted ductility of aluminium nanowires Oxidation can drastically change mechanical properties of nanostructures that typically have large surface-to-volume ratios. However, the underlying mechanisms describing the effect oxidation has on the mechanical properties of nanostructures have yet to be characterized. Here we use reactive molecular dynamics and show that the oxidation enhances the aluminium nanowire ductility, and the oxide shell exhibits superplastic behaviour. The oxide shell decreases the aluminium dislocation nucleation stress by increasing the activation volume and the number of nucleation sites. Superplasticity of the amorphous oxide shell is due to viscous flow as a result of healing of the broken aluminium–oxygen bonds by oxygen diffusion, below a critical strain rate. The interplay between the strain rate and oxidation rate is not only essential for designing nanodevices in ambient environments, but also controls interface properties in large-scale deformation processes. Nanowires (NWs) have attracted interest as potential building blocks for emerging electronic, optical and nanoelectromechanical devices due to their unique mechanical properties [1] , [2] , [3] , [4] . Nanoscale materials exhibit dramatically different deformation behaviour than their bulk counterparts. In situ transmission electron microscopy (TEM) [5] , [6] , [7] , [8] and molecular dynamics (MD) studies [9] , [10] , [11] , [12] , [13] showed that the plasticity of metallic NWs deformed under vacuum is controlled by the nucleation and escape of dislocations from the free surfaces, and required application of stresses a few orders of magnitude higher than necessary for the dislocation glide mechanisms of bulk crystalline materials. Alternatively, amorphous NWs may become superplastic at room temperature and can form long atomic chains at the fracture surfaces [14] , [15] . Consequently, statements such as ‘smaller is stronger’ [4] , [16] , [17] , [18] , [19] , [20] , ‘smaller is superplastic’ [14] , [15] , [21] or ‘smaller is softer’ [22] , have been used to describe mechanical properties of nanomaterials. In general, sophisticated tensile and compression tests of NWs were carried out in vacuum chambers, and thus, the effects of environment on their mechanical properties were not considered. As the surface-to-volume ratio increases, the influence of the oxidizing environment on the mechanical properties becomes more dominant. This effect is especially significant for technologically important lightweight metals such as Al, Mg and Ti, which have high oxygen affinity. Even under an ultrahigh vacuum, for example, at 10 −8 Torr sec O 2 (refs 23 , 24 ), an oxide layer can form on Al within seconds. According to our recent MD study [22] , a drastic decrease in the Young’s moduli of Al NWs (diameters below 100 nm) with decreasing NW diameters was predicted due to the formation of an amorphous oxide shell with a low modulus. In this study, the effects of simultaneous oxidation and deformation on the Al NWs’ properties, which present significant experimental challenges, are studied using MD simulations. The simulations are performed with a reactive force field (ReaxFF) [25] , [26] that accounts for charge transfer between aluminium and oxygen molecules. We show that the oxidation enhances the Al NW ductility. The oxide shell on the Al NW decreases the Al core’s dislocation nucleation stress by increasing both the activation volume and the number of nucleation sites. In an O 2 atmosphere, the amorphous oxide shell shows a superplastic behaviour as a result of viscous flow, in which oxygen diffusion heals the broken Al–O bonds, below a critical strain rate. We develop a model that explains the relationship between the strain rate and oxidation rate. These results demonstrate that understanding the environmental effects on the mechanical properties of NWs is important not only for developing nanoscale devices but also for increasing the efficiency of conventional manufacturing processes [27] , [28] , [29] , [30] . 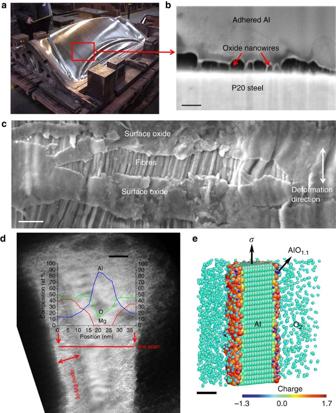Figure 1: Nanowire formation due to oxidation during bulk aluminium sheet forming process. (a) The outer surface of a stamping die made of P20 grade steel used to hot-form the lift gate made of Al-Mg Alloy, AA5083. (b) Cross-sectional FIB microstructure of the interface formed between the steel die surface and adhered Al (scale bar, 200 nm). (c) SEI of AA5083 alloy surface deformed at 723 K using a strain rate of 0.04 s−1showing fibre-like oxide structures (scale bar, 1 μm). (d) The cross-sectional high resolution TEM microstructure of an individual fibre that revealed its core shell (Al core, oxide shell) structure formed as a result of oxidation during deformation (scale bar, 10 nm). (e) The (100) cross-section of the nanowire model used to simulate the Al deformation and oxidation at the nanoscale. Al NWs were placed in an oxygen environment until an ~1-nm-thick AlO1.1layer formed on their surface. During the oxidation process electronic charge transferred from Al to O atoms yielded positively charged Al+1.5and O−1ions in the oxide layer, and formed a core shell nanowire structure with a metallic Al core and an oxide shell. Subsequently, the oxidized Al NWs were subjected to a tensile deformation in O2in the (001) direction (scale bar, 2 nm). Oxidized Al NW formation in hot forming and MD simulations Figure 1a shows an engineer holding a 30 cm long ruler standing next to an automobile lift gate steel (P20) mould that was used for hot stamping an Al-Mg alloy (AA5083) sheet at 723 K. The sliding contact at the interface induced material transfer from the Al-Mg alloy to the steel, which manifested itself in the form of fragments adhered to the mould surface [31] . The TEM cross-section of the adhered debris revealed that NWs (with diameters ranging from 20–50 nm) formed across the surfaces ( Fig. 1b ), akin to a miniature tensile sample. Interestingly, the composition of these NWs primarily consisted of oxides of Al and Mg [28] . The oxide NWs shown in Fig. 1b were uniformly elongated such that their lengths exceeded their diameters by more than 200%; therefore, they exhibited superplastic behaviour. NW oxides can also form on alloy surfaces during high-temperature deformation via the stretching of the oxide-rich surface covering the Al-Mg alloy surface ( Fig. 1c ), again showing long uniform elongation. An HR–TEM microstructure obtained from the NW cross-section revealed that each individual oxide NW had a core shell structure with an Al core covered with an oxide layer ( Fig. 1d ). This core (Al) shell (oxide) structure indicated that the NWs were formed as a result of dynamic oxidation during deformation. The formation of NWs promoted interfacial adhesion, which was detrimental to the forming process efficiency and Al surface quality. Figure 1: Nanowire formation due to oxidation during bulk aluminium sheet forming process. ( a ) The outer surface of a stamping die made of P20 grade steel used to hot-form the lift gate made of Al-Mg Alloy, AA5083. ( b ) Cross-sectional FIB microstructure of the interface formed between the steel die surface and adhered Al (scale bar, 200 nm). ( c ) SEI of AA5083 alloy surface deformed at 723 K using a strain rate of 0.04 s − 1 showing fibre-like oxide structures (scale bar, 1 μm). ( d ) The cross-sectional high resolution TEM microstructure of an individual fibre that revealed its core shell (Al core, oxide shell) structure formed as a result of oxidation during deformation (scale bar, 10 nm). ( e ) The (100) cross-section of the nanowire model used to simulate the Al deformation and oxidation at the nanoscale. Al NWs were placed in an oxygen environment until an ~1-nm-thick AlO 1.1 layer formed on their surface. During the oxidation process electronic charge transferred from Al to O atoms yielded positively charged Al +1.5 and O −1 ions in the oxide layer, and formed a core shell nanowire structure with a metallic Al core and an oxide shell. Subsequently, the oxidized Al NWs were subjected to a tensile deformation in O 2 in the (001) direction (scale bar, 2 nm). Full size image The NW morphology in Fig. 1d was used as the starting point for the MD simulations. A simulated single crystal Al NW (see ref. 22 for details) was oxidized at scaled room temperature (0.3 T m ) in a box containing high pressure of O 2 . As the oxidation of Al is a highly exothermic process, once O atoms react with Al atoms, an amorphous oxide structure forms on the surface. In this way, a core shell structured NW was formed, as shown in Fig. 1e . Al NW was shown to be covered by an ~1-nm-thick amorphous oxide layer (OC-Al NW) with an O/Al ratio of 1.1 and a Young's modulus of 25.5 GPa (ref. 22 ). The formation of an oxygen-deficient oxide structure is experimentally possible, as shown in previous observations, while ultrathin alumina films formed on NiAl reported to have AlO 1.3 stoichiometry as determined by STM and DFT [32] . An oxygen uptake rate of 30 g s −1 cm −2 (ref. 22 ) was calculated, which was 10–12 orders of magnitude higher than those experimentally observed. The typical strain rates [9] , [10] , [11] , [12] , [13] applied to NWs in MD studies were also 10–12 orders of magnitude higher than those determined experimentally so that the ratios of the simulated oxidation and strain rate were comparable with the experimental values, which allowed the interplay between the oxidation and strain rates to be captured. The oxidation simulations were purposely carried out at this high rate by using a high oxygen pressure (see Methods and ref. 22 ) to maintain this ratio. The OC-Al NWs were subjected to tensile strain using three different strain rates, 0.05% ps −1 (5 × 10 8 s −1 ), 0.5% ps −1 (5 × 10 8 s −1 ) and 5.0% ps −1 (5 × 10 10 s −1 ), in both vacuum and an O 2 environment (see Methods for details). Increased ductility observed in Al NWs deformed in O 2 The stress–strain curves of Al NW and OC-Al NWs obtained at a constant strain rate of 0.05% ps −1 are shown in Fig. 2a . The Al NW tested in vacuum ( Fig. 2a ) exhibited a high tensile (yield) strength followed by fracture at a low strain, while the OC-Al NW tested under the same conditions had a lower strength but significantly higher ductility. The greatest ductility was observed when the OC-Al NW was tested in O 2 indicating that the O 2 atmosphere drastically increased the NW's ductility. The pertinent mechanical properties of the NWs are shown in Table 1 . Al NWs tested under vacuum yielded at , which corresponded to a strain of . This was followed by a sudden drop in σ , and Al NW fractured at without necking, namely, in a quasi-brittle manner, as shown in Fig. 2b . The strength of OC-Al NW was initially controlled by the Al core that yielded at , but at a lower strain of than that of the Al NW’s. The oxide shell, however continued to deform after the fracture of the Al core at by viscous flow, and formed a neck around the Al fracture surface. For ε >20%, the oxide layer became thinner, and voids began to form and grow such that at ε =40% single atomic chains of Al–O were generated as shown in Fig. 2c . When OC-Al NW was deformed in O 2 , rather than in vacuum, its yield stress, controlled by the Al core, was smaller ( ); yet the deformation progressed at a constant stress by viscous flow of the oxide shell, which sustained a large strain of 78.0%, while exhibiting a uniform deformation without necking (as shown in Fig. 2d for ε =60.0%), which are characteristic features of superplastic deformation. 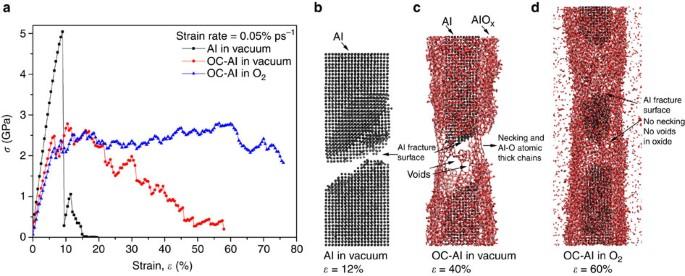Figure 2: Aluminium nanowire deformation in vacuum and O2environments. (a) A comparison of the stress–strain curves for Al and OC-Al NWs deformed under vacuum and in O2at a strain rate of 0.05% ps−1. (b) The atomic structure of Al NW fractured under vacuum atε=12% exhibited quasi-brittle fracture without necking. (c) OC-Al NW deformed under vacuum atε=40%. The fractured Al in the core and plastically deformed oxide at the surface formed Al–O chains and developed voids at the Al fracture surface. (d) OC-Al NW deformed in O2atε=60% showing that the Al core region was fractured and that the oxide deformed without any indication of a fracture or necking. Figure 2: Aluminium nanowire deformation in vacuum and O 2 environments. ( a ) A comparison of the stress–strain curves for Al and OC-Al NWs deformed under vacuum and in O 2 at a strain rate of 0.05% ps −1 . ( b ) The atomic structure of Al NW fractured under vacuum at ε =12% exhibited quasi-brittle fracture without necking. ( c ) OC-Al NW deformed under vacuum at ε =40%. The fractured Al in the core and plastically deformed oxide at the surface formed Al–O chains and developed voids at the Al fracture surface. ( d ) OC-Al NW deformed in O 2 at ε =60% showing that the Al core region was fractured and that the oxide deformed without any indication of a fracture or necking. Full size image Table 1 Mechanical properties of Al NWs deformed in vacuum and O 2 at different strain rates. Full size table Oxide shell enhanced the ductility of crystalline Al NWs The high yield strength and quasi-brittle fracture characteristics of Al NW deformed in vacuum were consistent with previous MD simulations [9] , [33] . 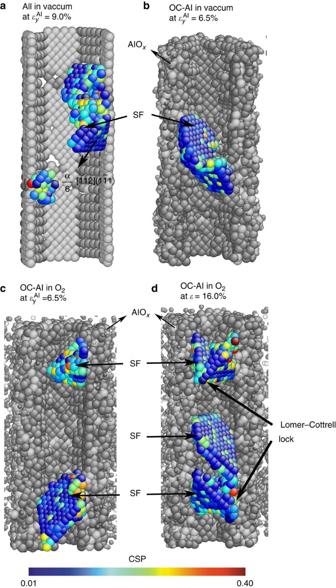Figure 3: SFs in aluminium deformed in vacuum and in O2at a strain rate of 0.05% ps−1. (a) SFs formed in Al NW deformed in vacuum at the yield point. (b) SFs formed in Al core of OC-Al NW deformed in vacuum at the yield point. (c) The SFs for an OC-Al NW deformed in O2at the yield point. (d) SFs formed in OC-Al NW deformed in O2atε=16%, indicating a Lomer–Cottrell lock formation. SFs were visualized using the CSP, where a CSP value of ~0.04 corresponds to an SF in the Al FCC lattice. Figure 3 provides details of dislocation initiation and glide mechanisms in the Al NW. The deformation mechanisms were investigated by determining the stacking faults (SFs) in the crystal using a centrosymmetry parameter [34] , [35] . Typically, the yielding of Al NW initiated by the nucleation of Shockley partial dislocations at the energetically favourable corners on the NW surface. Figure 3a shows details of two partial dislocations that nucleated from the intersection of (100) and (110) facets at the NW surface. These partial dislocations propagated by gliding on the slip system, where the maximum resolved shear stress occurred. The partials exited the NW surface, leaving an SF within the crystal and causing an abrupt stress release at ( Fig. 2a ). The Al NW fractured (at ) by cleavage that occurred along the (111) planes without nucleation of new dislocations. Figure 3: SFs in aluminium deformed in vacuum and in O 2 at a strain rate of 0.05% ps −1 . ( a ) SFs formed in Al NW deformed in vacuum at the yield point. ( b ) SFs formed in Al core of OC-Al NW deformed in vacuum at the yield point. ( c ) The SFs for an OC-Al NW deformed in O 2 at the yield point. ( d ) SFs formed in OC-Al NW deformed in O 2 at ε =16%, indicating a Lomer–Cottrell lock formation. SFs were visualized using the CSP, where a CSP value of ~0.04 corresponds to an SF in the Al FCC lattice. Full size image The surface oxide layer was responsible for both the decrease in the yield stress and the increase in the ductility of the Al NW. The disordered atomic structure of the Al/AlO x interface facilitated the nucleation of Shockley partial dislocations at the interface, hence easing the yielding of the Al core in OC-Al NW ( Fig. 3b ). The stress required for dislocation nucleation at a constant temperature ( T ) and strain rate ( ) was given as [36] , where corresponds to the athermal nucleation stress at 0 K, Q* is the activation energy barrier for the dislocation nucleation in the absence of stress, is the activation volume, k B is the Boltzmann constant, N is the number of nucleation sites, v 0 is the atomic vibrational frequency and E is the Young’s modulus. The linear regression analysis of versus (according to the values listed in Table 1 ) gives the slope, and the intercept, . From the slope values, was obtained for the Al-NW,—in agreement with values of 1–10 b 3 (ref. 36 ) reported for surface dislocation nucleation in nanostructures under vacuum. The oxide shell increased the dislocation nucleation activation volume ~4 times, as for OC-Al NW an (under vacuum), and an (in O 2 ) were calculated, thus lowering the yield stress of the Al core. The values of OC-Al-NW were significantly lower than that of a bulk dislocation nucleation (100–1,000 b 3 ), for example, for Frank–Read sources. When the OC-Al NW was deformed under an O 2 atmosphere, the nucleation of Shockley partials occurred at the Al/AlO x interface ( Fig. 3c ) at the same activation volume, but a drastic increase in the number of dislocation nucleation events were noted, as evident by the increased number of SFs in the Al at ε =16.0% in Fig. 3d . For OC-Al NW, the activation energy of dislocation nucleation depends strongly on the nature of interface structure (Al/AlO x ), where it is reasonable to assume that Q* and do not change with the environment. The ratio of N in the two environments can also be computed from the intercept of linear fitting of the σ versus . The calculated N values for OC-Al NW were ~7 times greater in O 2 compared with vacuum, thus causing further decrease in the yield strength for the OC-Al-NW ( Fig. 2a ). Consequently, the frequency of dislocation–dislocation interactions that occurred within the Al increased considerably. Figure 3d shows a couple of examples of two SFs meeting at an angle of 70.5° to form Lomer–Cottrell locks. Lomer–Cottrell lock formation in nanocrystalline Al deformed under vacuum was found in previous MD studies but for larger size samples consisting of 20–70 nm grains [37] . The Lomer–Cottrell locks restricted the dislocation mobility, and thus caused an increase in the strength of the crystal between ε =14.0–16.0% by 0.23 GPa. Dislocations inside a NW would readily escape from the free surface due to the image forces acting on them [38] . On the other hand, dislocations can only escape through the Al/AlO x interface if the oxide layer had a lower shear modulus, , than Al [38] , [39] , μ Al . Our recent work demonstrated that the oxide shell had in fact a lower Young’s modulus of ( ) than Al with E Al =61.2 GPa ( μ Al =23.54 GPa) [22] . The image forces, F , acting on a dislocation in the vicinity of free Al surface and near the Al/AlO x interface were estimated using the relation (ref. 39 ), where, μ Al is the shear modulus of Al, R is the effective modulus (See Methods section for details) for Al, and r is the distance from the dislocation to its nearest image, which has a minimum value r= 2 b . Accordingly, the maximum image forces under vacuum were N m −1 for an Al NW surface and N m −1 near the Al/AlO x interface. Consequently, as , the dislocation escape would be hindered in OC-Al NW, and this prolonged dislocations mobility within the Al core improving its ductility of (note that the fracture strain of OC-Al NW is higher than Al NW when tested in vacuum, Fig. 2 and Table 1 ). Superplasticity of the amorphous oxide shell deformed in O 2 The AlO x shell deformed by the collective diffusion of Al and O atoms in the direction of the applied strain in both vacuum and O 2 environments. 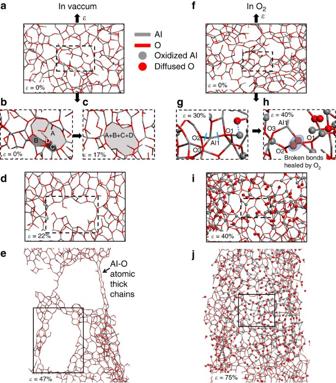Figure 4: Deformation mechanisms of the amorphous oxide under vacuum and O2. (a–e) The changes in the amorphous structure of the oxide deformed under vacuum and (f–j) in O2. For vacuum, (b,c) shows the formation of voids due to Al–O bonds breaking and generation of larger rings at the expense of smaller rings. (d,e) Further deformation yielded larger voids and formed atomic Al–O chains at the fracture surface. (g,h) shows that when stretched in an O2atmosphere, O atoms diffused throughout the oxide structure and attached to the broken Al–O chains, which has a healing effect that allowed for repairing of bonds broken during applied strain and led to superplastic deformation suppressing the void formation (i,j). Figure 4 illustrates the deformation mechanisms of the oxide layer stretched in both vacuum ( Fig. 4a–e ) and O 2 ( Fig. 4f–j ). Under vacuum, the Al–O rings opened with the applied strain ( Fig. 4a ). Fracture was initiated when the weaker homopolar O–O bonds broke, followed by breaking of the Al–O bonds. The Al–O rings then expanded at the expense of smaller rings and formed the voids shown in ( Fig. 4b,c ), in accordance with the increase in the free volume increase during elongation. These voids enlarged further with the increasing strain ( Fig. 4d ), and eventually formed Al–O-Al atomic chains ( Fig. 4e ) at the neck ( Fig. 2c ). When OC-Al NW was tested under an O 2 atmosphere ( Fig. 4f ), the O 2 diffused to the surface of NW was chemisorbed to the broken Al–O bonds at the surface ( Fig. 4g ) and initially formed an Al–O–O bond ( Fig. 4h ). These weak homopolar O–O bonds were then broken at a higher strain with one O atom becoming connected to nearby Al atoms ( Fig. 4i ). This mechanism ‘healed’ the Al–O bond network. As this healing process continued, the length of OC-Al NW extended uniformly to large strains without fracture or necking. As a result, no large rings formed in the structure stretched under O 2 ( Fig. 4j ). A statistical analysis of the voids that formed between the Al–O rings (at Δε=0.4, as shown in Supplementary Fig. 1 ) supported opposite Al–O ring evolution patterns under vacuum and in O 2 . Under vacuum, the number of large Al–O rings (with 16, 18, 20 and 24 atoms) increased at the expense of smaller rings (with 4, 10, 12 and 14 atoms), in conjunction with void formation. In contrast, in O 2 , the number of larger rings (with 10, 12 and 14 atoms) decreased and the number of smaller, 4 atoms, Al–O rings increased due to the healing effect of O 2 diffused into the oxide phase. Figure 4: Deformation mechanisms of the amorphous oxide under vacuum and O 2 . ( a – e ) The changes in the amorphous structure of the oxide deformed under vacuum and ( f – j ) in O 2 . For vacuum, ( b , c ) shows the formation of voids due to Al–O bonds breaking and generation of larger rings at the expense of smaller rings. ( d , e ) Further deformation yielded larger voids and formed atomic Al–O chains at the fracture surface. ( g , h ) shows that when stretched in an O 2 atmosphere, O atoms diffused throughout the oxide structure and attached to the broken Al–O chains, which has a healing effect that allowed for repairing of bonds broken during applied strain and led to superplastic deformation suppressing the void formation ( i , j ). Full size image Continuous O 2 diffusion promoted superplastic deformation of the oxide shell on the OC-Al NW tested in the O 2 environment, as shown in Fig. 2d for a strain rate of 0.05% ps −1 . At this low strain rate, sufficient time was available for diffusing oxygen atoms to repair the broken Al–O bonds, and prevented necking formation ( Fig. 2d ). Therefore, for a particular oxidation rate during elongation, there should be a critical strain rate, ε c , below which OC-Al NW would demonstrate superplasticity. The decrease in the thickness during deformation was compensated for the increased oxide thickness due to O 2 diffusion, and as shown before, the oxide thickness remained constant regardless of the applied strain ( Fig. 2d ). Accordingly, for an initial oxide thickness of x 0 , assuming that the application of a strain of ε per unit time would cause a reduction in the oxide thickness, Δ x , that is compensated by the oxidation process. Assuming a linear oxidation rate [40] , yields the following: By combining equations (1) and (2) and using the expression for C provided in a diffusion controlled growth model [40] , can be expressed as follows: where h is the rate constant at the gas-oxide interface, k is the rate constant at the Al–oxide interface, K is Henry’s law constant, is the O 2 partial pressure, and is the number of oxygen molecules incorporated into a unit volume of the oxide layer [40] . Both rate constants h and k will increase with temperature ( T ) as they obey an Arrhenius-type relationship. Therefore, superplastic oxides become easier to observe at a higher temperature and oxygen rich environment, as increases with increasing T and . The oxide thickness, x 0 was reported to remain at a constant value of ~3.8 nm for Al nanopowders with diameters larger than 20 nm [41] , [42] . This means, equation (3) is expected to be size independent only when the contribution of the thin oxide layer to the total deformation of Al is small and x 0 remains a constant in large-sized samples [22] . However, at the nanoscale, when x 0 decreases with the size of the Al [41] , [42] , without considering any other size-dependent properties, such as oxidation rates, will increase with decreasing size, so that it will be easier to deform superplasticity in smaller Al NWs. Assuming a constant oxide density of 2.78 g cm −3 , Δ x was estimated from the number of Al and O atoms in the oxide per unit of time for the last 20 ps of the oxidation process [22] , as C =4.48 × 10 −4 nm ps −1 . Thus, the critical strain rate of was calculated based on equation (3). MD simulations performed using higher strain rates of 0.5% ps −1 and 5.0% ps −1 confirmed that for strain rates above oxide did not show superplastic behaviour, and the stress–strain curve of the OC-Al-NW in O 2 was similar to that under vacuum, as shown in Fig. 5a . In other words, the strain rate did not significantly affect the U plastic of Al and OC-Al NWs, when deformed under vacuum; however, the U plastic decreased with the increasing strain rate, such that at % ps −1 , the U plastic values for OC-Al NW under vacuum and in O 2 were similar ( Table 1 ). At , U plastic was twice that in O 2 relative to vacuum ( Table 1 ). An atomistic argument for the above model can be given by considering the number of atoms in the oxide layer ( Supplementary Fig. 2 ) indicates that more Al and O atoms grew into the oxide layer, when OC-Al-NW was deformed in O 2 at a low strain rate of 0.05% ps −1 , whereas the O/Al ratio remained constant even at high strain. In contrast, under the vacuum condition, the O/Al ratio decreased during stretching (see Supplementary Fig. 3 and Supplementary Discussion). 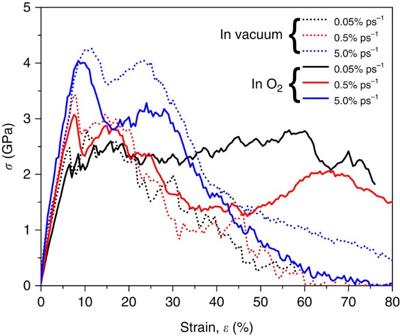Figure 5: Stress–strain curves for OC-Al NW deformed in vacuum and O2at different strain rates. At high strain rates, the stress–strain curves in O2are similar to those in vacuum. Figure 5: Stress–strain curves for OC-Al NW deformed in vacuum and O 2 at different strain rates. At high strain rates, the stress–strain curves in O 2 are similar to those in vacuum. Full size image Equation (3) can be used to determine from experimentally obtained oxidation data [40] . For example, using the values in ref. 43 where an oxidation rate C =7.46 × 10 −5 nm s −1 was measured at 673 K ( ) for pure Al using an oxide thickness of x 0 =1 nm, a critical strain rate of s − 1 can be determined. Observations made on the fresh fracture surfaces of Al alloys, subjected to tensile deformation showed that oxide fibres were formed superplastically at s − 1 as a result of dynamic oxidation [29] , [30] , [31] . In addition, interfaces between a bulk Al sheet surface and a counterface were shown to exhibit oxide fibres that clearly exhibited such superplastic behaviour as shown in Fig. 1 . The critical strain rate, below which superplastic fibres form, is expected to vary with alloy compositions, temperature and gas environment in agreement with current model between 10 − 3 and 10 − 5 s − 1 (ref. 30 ). In summary, this work demonstrated that nanosized native oxide of Al significantly enhanced the ductility of Al NWs. Not only did the dislocation activity in the Al crystal increase, but when tested in an O 2 atmosphere, the oxide shell also showed superplasticity. Al–O rings and Al–O atomic chains were observed at the fracture surface, which suggested both that one- and two-dimensional oxide structures can be produced by subjecting the oxide to tensile deformation and that the properties of these structures could be modified in an O 2 environment. These results for the nanoscale also advised that large-scale adhesion problems during Al manufacturing due to the superplastic deformation of the oxide can be controlled by removing oxygen from the environment (using an inert atmosphere). Consequently, one can tailor the atmospheric conditions to alter the nanoscale mechanical properties of materials to improve their manufacturing processes at industrial scale. The use of a ReaxFF that can predict the Al stacking fault energy and melting temperature more accurately would enable a more precise depiction of the deformation mechanisms of Al, and the interaction of dislocations with oxygen impurities or oxide shell would be made possible. Hot-forming experiments High-temperature tensile tests were carried out using an instrumented hot forming simulator (also functions as a tribometer) designed and developed at the University of Windsor to apply uniaxial tensile stresses at constant strain rates and temperatures as described in ref. 29 . AA5083 strips (H18) (5.0 mm wide) were tested at a temperature of 723 K and strain rate of 0.04 s −1 . One surface of the AA5083 strip (along the rolling direction) was put in sliding contact with P20 grade tool steel pin. The material transferred from AA5083 to pin surface during sliding contact was studied. AA5083 strip was tested in the as received condition, that is, without removing the surface oxide formed during prior processing. Microstructure of adhered interface A JEOL 840 SEM and a ZEISS NVision 40 CrossBeam workstation (focused ion beam (FIB)), were used to investigate microstructures at the interface formed between the AA5083 and P20 steel. The cross-sectional microstructure shown in Fig. 1b was prepared by FIB milling. Care was taken to avoid ion beam damage to the surface by depositing a layer of carbon. A trench was milled, using a Ga + ion beam at an accelerating voltage of 30 kV with beam currents ranging from 13 nA to 700 pA. Final polishing was done at a low voltage of 5 kV and ion beam current of 80 pA to minimize the beam damage on the specimen. Cross-sectional trenches from AA5083 deformed surfaces were also ion milled on the deformed surface oxide layers shown in Fig. 1c ; along the oxide fibres generated during high-temperature deformation and site-specific TEM samples were prepared by FIB lift-out method from selected fibres. The microstructure of a single oxide fibre ( Fig. 1d ) was taken using a JEOL JEM-2100F field emission TEM operated at 200 kV. The superimposed electron dispersive X-ray spectroscopy scans in Fig. 1d were obtained using an EDAX system. MD simulations A ReaxFF, namely, ReaxFF, was used for MD simulations as implemented [44] in LAMMPS [45] to study the oxidation and deformation of aluminium simultaneously. In ReaxFF, the total energy of the system is defined as being composed of bonding, Columbic, over-coordination and van der Waals energies, and the Coulomb energy calculations determine the charge of each atom in every MD step via an electron equilibration method [46] . All MD calculations were performed at a constant temperature of T =200 K using a Nose–Hoover thermostat [47] , [48] . ReaxFF predicted the melting temperature ( T m (MD)) of Al as 600 K, lower than the experimental value ( T m (exp)=933K). So all the MD simulations were performed at a scale room temperature, 0.3 T m (MD) or 200 K. The effect of oxidation on the Al deformation was investigated in two steps. First, a 4.0 nm diameter and 10.2 nm long Al nanowire was constructed with a faceted cross-section composed of {100} and {110} surfaces containing 8,500 Al atoms. This Al nanowire was periodic in the [001] direction and placed in a box containing 4,000 O 2 molecules with a density 188 times that of ambient conditions. After a 50 ps oxidation, a 0.9 nm thick amorphous oxide layer passivated the Al nanowire surface with a stoichiometry of AlO 1.1 . In deformation simulations, tensile strain was applied in the [001] direction at increments of 0.5% and the structure was allowed to relax at each strain increment. The strain rate was changed using different relaxation times between consecutive strain increments. Three strain rates were used, namely, 0.05% ps − 1 (5 × 10 8 s −1 ), 0.5% ps − 1 (5 × 10 8 s −1 ) and 5.0% ps − 1 (5 × 10 10 s − 1 ). The strain was applied until the nanowire fractured. The virial theorem was used to obtain the engineering stress–strain curve in the [001] direction. Based on this simulated stress–strain curve, the yield stress, σ y , at the yield strain, ε y , was defined as the maximum stress before a dislocation nucleation occurred in Al, after which a drop in σ was observed. The plastic energy ( U plastic ) and elastic energy ( U elastic ) were estimated from the area under the stress–strain curves. U elastic was calculated for , and U plastic was calculated for either to the strain at fracture of NW or formation of an atomically thick Al–O chain. The definition of a centrosymmetry parameter [34] as implemented by the ATOMEYE [35] programme was used to visualize the aluminium SFs. Plastic deformation in the amorphous AlO x was revealed by the changes in the Al–O bond structure, and the statistical analysis of shortest path rings [49] were calculated using the R.I.N.G.S. code [50] . Calculation of image force acting on a dislocation The image force per unit length between a screw dislocation with a burgers vector, b , within crystal B and its nearest image in crystal A was calculated as according to Koehler [39] , where , μ A and μ B are the shear modulus of metals A and B, respectively, and r is the distance between the dislocation and its nearest image. This formula was used to calculate the maximum image force acting on a partial dislocation when r =2 b with a Burger’s vector of within the Al crystal and with a lattice parameter of a =4.05 Å near the Al/AlO x interface. In our system, and μ B = μ Al , and we estimated the modulus of rigidity for Al and AlO x from the calculated Young’s modulus (E) using . Here, we assumed the Poisson ratio ( ) as 0.3 for Al and 0.15 for AlO x . How to cite this article : Sen, F. G. et al . Oxidation-assisted ductility in aluminium nanowires. Nat. Commun. 5:3959 doi: 10.1038/ncomms4959 (2014).